Larval dispersal drives trophic structure across Pacific coral reefs Top predators are a critical part of healthy ecosystems. Yet, these species are often absent from spatially isolated habitats leading to the pervasive view that fragmented ecological communities collapse from the top down. Here we study reef fish from coral reef communities across the Pacific Ocean. Our analysis shows that species richness of reef fish top predators is relatively stable across habitats that vary widely in spatial isolation and total species richness. In contrast, species richness of prey reef fish declines rapidly with increasing isolation. By consequence, species-poor communities from isolated islands have three times as many predator species per prey species as near-shore communities. We develop and test a colonization–extinction model to reveal how larval dispersal patterns shape this ocean-scale gradient in trophic structure. Top predators are often conspicuously absent from isolated habitats [1] , [2] , [3] , [4] , [5] , [6] , [7] , [8] . Explanations for such spatial variation in trophic structure are numerous: predators often have greater resource requirements [9] , [10] , [11] , larger body sizes [12] , smaller population sizes [13] and slower population growth rates [14] than species lower in the food web. Moreover, in some ecosystems, predators are poorer dispersers than their prey, making it less likely that they will colonize isolated habitats, let alone persist there [1] , [15] . In marine systems, however, genetic estimates of dispersal distances provide some evidence that species higher in the food web disperse more widely than species in lower trophic levels [16] . If predators disperse widely, serial influx of colonists could rescue isolated predator populations from extinction. An immediate question, then, is how do differences in the dispersal patterns of predators and their prey affect geographic patterns of community trophic structure? To answer this question, we analysed a database of published species lists from 35 major coral reef fish communities across the Pacific Ocean consisting of 1,350 total species. Using diet and life history information, we classified each species as either a piscivorous top predator (hereafter predator) or as a species lower on the food chain (hereafter prey). The ratio of the number of predator species to the number of prey species (predator–prey ratio [17] , R ; Fig. 1 , circle colour) and total reef fish species richness (circle size) vary widely among Pacific coral reef communities. Total reef fish species richness decreases with increasing isolation as in other systems [18] , [19] and predator–prey ratio varies among islands by a factor of 3 (range: 0.34–1.1 predator species per prey species; Fig. 1 ). However, in stark contrast to patterns reported from other ecosystems [20] , the coral reef communities with the highest predator–prey ratios are species-poor communities from the most isolated habitats (for example, Midway, Tuvalu; Fig. 1 inset), whereas communities located near large landmasses (for example, Palau, Vanuatu) have high total species richness and low predator–prey ratios. 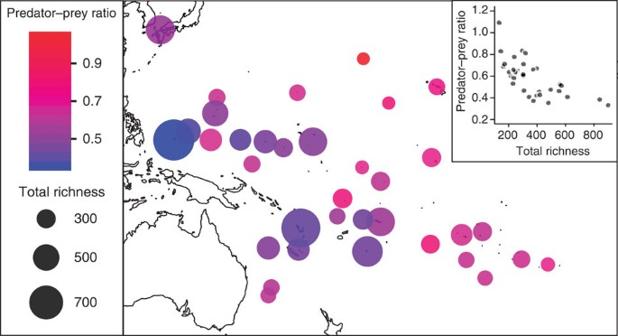Figure 1: Predator–prey ratio and total species richness in coral reef fish communities from 35 Pacific habitats. Circle size increases with increasing total species richness (# of predator species+# of prey species); colour indicates low (blue) or high (red) predator–prey ratio. Inset showing that predator–prey ratio decreases strongly with increasing total species richness. Figure 1: Predator–prey ratio and total species richness in coral reef fish communities from 35 Pacific habitats. Circle size increases with increasing total species richness (# of predator species+# of prey species); colour indicates low (blue) or high (red) predator–prey ratio. Inset showing that predator–prey ratio decreases strongly with increasing total species richness. Full size image Two features of Pacific coral reef communities are at odds with theory and observations from other systems. First, predator–prey ratio is high in isolated communities and low in proximate ones. Second, predator–prey ratio is negatively correlated with total reef fish species richness ( Fig. 1 , inset) instead of being positively correlated with, or invariant of total richness as in many terrestrial and aquatic ecosystems [20] . These findings contradict theoretical predictions [13] , [21] and empirical studies of other ecosystems, which suggest that species highest in the food web should be most sensitive to habitat isolation [4] , [10] , [12] , [22] . Here we develop a mathematical dispersal–colonization–extinction framework that resolves both of these discrepancies. The framework models species composition in a given habitat as an equilibrium between colonization of new species and extinction of those already present [23] , but builds on this concept by incorporating a basic life history trait of reef fish, the duration of pelagic (open ocean) larval dispersal, which can influence species’ dispersal distances [24] . We model larval dispersal to predict colonization rate at focal reefs, and use colonization rate to predict how species richness and predator–prey ratio vary across space. Modelling framework Most reef fishes exhibit a multi-stage lifecycle involving a dispersive larval stage, followed by a non-dispersive adult stage. The length of time larvae spend in the dispersive stage is known as pelagic larval duration (PLD). Limited dispersal due to limited PLD has been proposed to explain why total reef fish species richness is lower in more isolated habitats and why species that do occur in isolated habitats have higher mean PLD than those inhabiting near-shore habitats [18] , [25] . In general, short-term estimates of dispersal distance are positively correlated with PLD among marine species, although the strength of this relationship varies across the range of PLDs [26] . In this study, we are most interested in dispersal that allows species to colonize new habitats over long ecological timescales (that is, hundreds to thousands of fish generations). Genetic estimates of dispersal distances may provide the best available indices of dispersal distance on such timescales. Genetic estimates of dispersal distance are strongly correlated with PLD, and also agree reasonably well with dispersal distance estimates from computational Lagrangian particle models, which assume that marine larvae disperse like passive particles through the plankton [24] . Here we take an analytical approach that includes PLD along with other basic features of the larval dispersal process. To relate PLD to dispersal and colonization rates of predators and prey, we use a diffusion–advection–mortality model [27] , which describes dispersal of fish larvae from large source populations ( Figs 2 , 3 ; full model described in Supplementary Methods ). 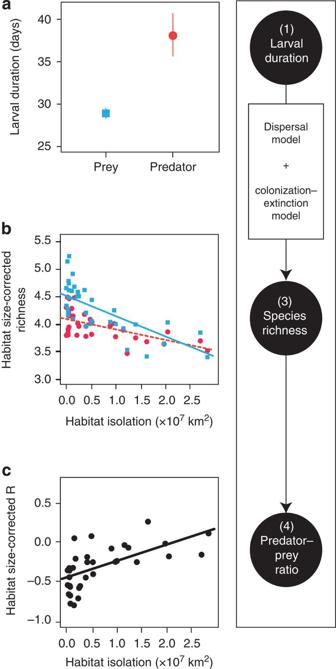Figure 2: Integration of dispersal model with colonization–extinction model and fitting of model to Pacific reef fish data. (a) Larval duration data indicate that predators (red) have longer mean PLD than prey (blue;τprey=(28.3, 29.5) days,τpred=38.1 (35.6, 40.7) days, mean number of days (lower, upper s.e.m.);t-test:t=3.92,P<0.001,nprey=347,npredators=35, means and s.e. back-transformed from log scale). (b) Model predicts that predators’ longer larval durations (τpred>τprey) will cause a relatively shallow decay of predator richness (red) compared with relatively rapid decay of prey richness (blue) with increasing habitat isolation. (c) Mechanistic model of predator–prey ratio fitted to data. Model predicts that the predator–prey ratio (R) increases with habitat isolation, measured as squared distance from the focal site to the nearest landmass with area >104km2(see Methods for statistics). Predictions are robust to other metrics of isolation. The ratio of predator colonization rate ( C pred ) to prey colonization rate ( C prey ) at a given location obeys Figure 2: Integration of dispersal model with colonization–extinction model and fitting of model to Pacific reef fish data. ( a ) Larval duration data indicate that predators (red) have longer mean PLD than prey (blue; τ prey =(28.3, 29.5) days, τ pred =38.1 (35.6, 40.7) days, mean number of days (lower, upper s.e.m. ); t -test: t =3.92, P <0.001, n prey=347, n predators=35, means and s.e. back-transformed from log scale). ( b ) Model predicts that predators’ longer larval durations ( τ pred > τ prey ) will cause a relatively shallow decay of predator richness (red) compared with relatively rapid decay of prey richness (blue) with increasing habitat isolation. ( c ) Mechanistic model of predator–prey ratio fitted to data. Model predicts that the predator–prey ratio ( R ) increases with habitat isolation, measured as squared distance from the focal site to the nearest landmass with area >10 4 km 2 (see Methods for statistics). Predictions are robust to other metrics of isolation. 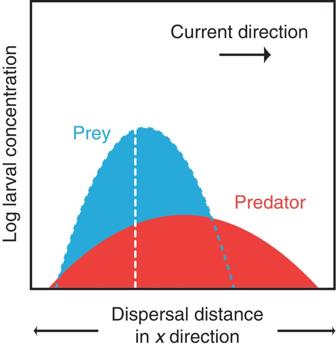Figure 3: Diagram illustrating differential spreading of predator larvae. Larval concentration of a species of predator (red) and prey (blue) at different distances from a source population (dashed vertical white line), given that predator spends more time dispersing than prey. Larval dispersal is modelled using a diffusion–advection–mortality model. Larvae originate at a source location and larval concentration,Iiof prey (i=1) or predators (i=2) is governed by the equation,, in two dimension (2D; Δ is 2D Laplacian,uandvare mean speeds of advective currents inxandydirections, respectively,σrepresents the effective diffusivity of larvae andμiis mortality rate)27. Full size image Figure 3: Diagram illustrating differential spreading of predator larvae. Larval concentration of a species of predator (red) and prey (blue) at different distances from a source population (dashed vertical white line), given that predator spends more time dispersing than prey. Larval dispersal is modelled using a diffusion–advection–mortality model. Larvae originate at a source location and larval concentration, I i of prey ( i =1) or predators ( i =2) is governed by the equation, , in two dimension (2D; Δ is 2D Laplacian, u and v are mean speeds of advective currents in x and y directions, respectively, σ represents the effective diffusivity of larvae and μ i is mortality rate) [27] . Full size image where τ pred is predator PLD, τ prey is prey PLD, d is the distance between the source of larvae and the focal habitat and σ ( σ >0) is the effective diffusivity of predator and prey larvae during dispersal. The ratio of predator larvae to prey larvae colonizing a site will increase with increasing habitat isolation if predators spend more time drifting in the plankton than their prey (that is, τ pred > τ prey ). This is because a longer PLD causes predator larvae to spread farther from their point of release ( Fig. 3 ), creating a distribution of predator larvae that is spread more uniformly over space than the distribution of prey larvae ( Supplementary Methods section 4.1 and Supplementary Fig. 2 discuss multiple larval sources). Data from 382 species of Indo–Pacific reef-associated fish from a recently published database [28] ( Supplementary Data 1 ; n prey=347, n predators=35) indicate that mean predator PLD is 28% longer than mean prey PLD ( Fig. 2a ). Equation (1) therefore predicts that the ratio of predator to prey colonization rates should increase with increasing habitat isolation. To connect colonization rates with standing species richness and predator–prey ratio, we use a colonization–extinction model [23] ( Fig. 2b,c ). In keeping with classical models [13] , we assume that species within each trophic level colonize and go extinct from habitats identically and independently. We calculate the predator–prey ratio R in a focal habitat as the ratio of the equilibrium number of predator species ( S pred ) to the equilibrium number of prey species ( S prey ), , where and are the equilibrium probabilities that any given predator or prey species occur in the community ( Supplementary Methods ). The dynamics of p pred and p prey can be modelled by the differential equations, and , with equilibrium , where the subscript i denotes predators or prey and C i and E i denote colonization and extinction rates, respectively [13] (we discuss coupling between predators and prey in Supplementary Methods ). When the equilibrium occurrence probability of any given species is small, Predator–prey ratio is proportional to the ratio of predator to prey colonization rates, which may vary with habitat isolation, and proportional to the ratio of extinction rates, which will not generally depend directly on habitat isolation. Combining the model of larval dispersal described above (equation (1)) with the equilibrium model for predator–prey ratio (equation (2)) shows how predator–prey ratio depends on habitat isolation: where r 0 and r 1 are positive constants that capture factors that do not depend on isolation (for example, differential larval production, differential extinction rates and larval mortality rates). Equation (3) states that predator–prey ratio should increase with increasing isolation distance when predator PLD is longer than prey PLD (that is, τ pred > τ prey ). It also predicts the form of the function relating isolation distance, d , to predator–prey ratio, R . Below we describe how this predicted functional form can be fit to data, and explore whether the model developed above can account for patterns evident in the Pacific reef fish data. Fitting models to data By log (ln) transforming both sides of equation (3), we can fit the predicted function of ln( R ) as a linear function of d 2 directly to the predator–prey ratio data shown in Fig. 1 (fit shown in Fig. 2c , statistical models and spatial autocorrelation discussed in Methods). In what follows, we will refer to d 2 as ‘habitat isolation’ and d as ‘isolation distance’. Figure 2c shows that predator–prey ratio increases with increasing habitat isolation as predicted by our model ( P =1.8 × 10 −4 ; habitat isolation measured as squared distance to nearest landmass with area >10 4 km 2 ; other isolation metrics yield similar results; Supplementary Methods ). This occurs because predator richness ( Fig. 2b , red circles, dashed line) is less sensitive to habitat isolation than is prey richness ( Fig. 2b , blue squares, solid line, P =9.5 × 10 −6 , r 2 =0.78) as our model predicts, given that predators have longer PLDs than prey ( Fig. 2a ). The model thus resolves the first discrepancy between observations from other ecosystems and our observations from coral reef communities, that isolated reef communities have the highest predator–prey ratios. Isolated communities have high predator–prey ratios because at their times of settlement, predator larvae are spread more uniformly across space than prey larvae. This makes predator larval supply ( Fig. 3 ), colonization rate and, consequently, species richness ( Fig. 2b ) relatively insensitive to habitat isolation. Prey richness falls more rapidly with increasing habitat isolation causing predator–prey ratio to rise as isolation increases ( Fig. 2c ). A second prediction follows from the form of the functions relating S pred and S prey to habitat isolation. When currents spread larvae but directional advection is weak, our model predicts that the richness of species in trophic group i is , where K i is a trophic level-specific constant ( Supplementary Methods ). Substituting this expression for prey richness into the corresponding expression for predator richness reveals that ; predator richness should be a power function of prey richness with exponent λ = τ prey / τ pred . 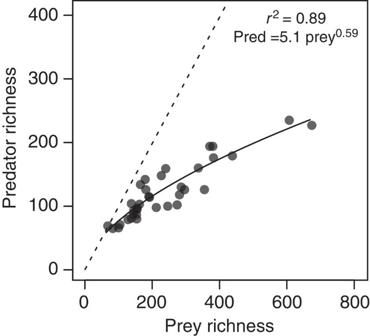Figure 4: Relationship between reef fish prey and predator species richness in Pacific coral reef communities. Functional form (power function) predicted from dispersal–colonization–extinction framework and fitted using generalized nonlinear least squares accounting for spatial autocorrelation. Data from 35 islands across the Pacific (1,350 total species). Figure 4 shows this predicted function fitted to the Pacific reef fish data. Communities with higher total richness (that is, points closer to the upper right corner of Fig. 4 ) are farther from the dashed one-to-one line. As predicted, the relationship between S pred and S prey is described well by a power function (exponent=0.59, 95% confidence interval (CI)=(0.5, 0.68), P =4.9 × 10 −16 , r 2 =0.89); a power function provides better prediction of the data than the linear function that would result if predator–prey ratio were constant (Akaike’s Information Criterion (AIC) power model: 313; AIC linear model: 317), which is consistent with the observation that predator–prey ratio declines as total species richness increases ( Fig. 1 , inset). Because the power function exponent λ is determined solely by predator and prey PLDs, we can independently estimate λ from the PLD data shown in Fig. 2a . Dividing mean prey PLD by mean predator PLD indicates that λ =0.77 (delta method 95% CI=(0.65, 0.88)), close to the fitted value of 0.59 (0.5, 0.68), particularly considering that the former ignores effects of prevailing directional currents on dispersal patterns. Critically, both predicted and observed exponents are less than 1. The model correctly predicts that communities with low overall richness will have the highest predator–prey ratios, resolving the second discrepancy between patterns of predator–prey ratio in other ecosystems and patterns in Pacific coral reef communities. Figure 4: Relationship between reef fish prey and predator species richness in Pacific coral reef communities. Functional form (power function) predicted from dispersal–colonization–extinction framework and fitted using generalized nonlinear least squares accounting for spatial autocorrelation. Data from 35 islands across the Pacific (1,350 total species). Full size image The qualitative predictions of our model are robust to changes in our assumptions about reef fish dispersal and colonization. For example, the simplified model of colonization–extinction dynamics of equation (2) does not account for the dependence of predators on the presence of their prey [9] , [10] , [11] . Incorporating this prey dependence ( Supplementary Methods ) shows that the predator–prey ratio R can still increase with habitat isolation in a manner consistent with equation (3) for a range of habitat isolation values. The coupled predator–prey colonization–extinction model developed in Supplementary Methods reveals that predator diet specialization also affects the relationship between predator–prey ratio and habitat isolation. If predators are highly specialized, predator–prey ratio will initially increase as habitat isolation increases, but will quickly begin to decline as the prey of specialist predators disappear from isolated habitats, and predators are thereby driven extinct. However, when predators are generalists as in the case of many reef fish predators [29] , R will continue to increase with habitat isolation over a wide range of isolation values as observed in the Pacific reef fish data. Intuitively, this is because generalist predators can persist on a wide range of different prey and the absence or loss of prey from isolated habitats only affects a predator if all of that predator’s prey species are simultaneously absent. The coupling between predator and prey richness will be even weaker if predators can persist by eating juvenile conspecifics and juveniles of other piscivorous species [29] . In the extreme case where predators eat juveniles of all species, the coupling between predator and prey equations becomes very weak and the uncoupled equations presented above are approximately recovered ( Supplementary Methods ). Processes other than those described by our model undoubtedly contribute to the variation present in Figs 1 , 2b,c and 4 . We do not consider effects of predators on prey extinction [30] , [31] , [32] , effects of complex trophic structure [10] , local speciation [33] , other life history characteristics such as body size, diurnal or nocturnal activity and schooling behaviour [28] , nor do we consider complex ocean currents [34] . The amount of population self-recruitment, post-arrival establishment success and species body sizes may differ among predators and prey [28] , leading to differences in predator and prey extinction rates (equation (2)). However, these differences will not affect the isolation dependence of predator–prey ratio (that is, they affect r 1 only in equation (3)) unless they generate a correlation between extinction rate and habitat isolation. Because we are interested in the isolation dependence of the predator–prey ratio, we do not consider these factors explicitly. Previous studies have noted that selective overharvesting of top predators may compound effects of habitat loss on predator richness [8] . In marine ecosystems, disproportionate fishing pressure on top predators (that is, ‘fishing down food webs’) is well documented [35] , [36] , [37] , although local anthropogenic extinctions are seldom described in reef fish systems. In Supplementary Methods , we explore whether fishing pressure on top predators alone can account for the patterns of reef fish predator–prey ratio described above. Statistical models that contain indices of fishing pressure but lack the functional relationship between predator–prey ratio and habitat isolation derived above provide a poor fit to data. Overfishing of top predators alone does not account for the patterns reported here. Mounting evidence suggests that species’ dispersal patterns shape community and food web structure in many ecosystems [38] , [39] , [40] , [41] , [42] . For example, competing reef fish species in the Great Barrier Reef ecosystem appear to have different dispersal abilities, and this difference may explain the complex patterns of species coexistence observed across the Great Barrier Reef [40] . Dispersal has also been implicated as a potential cause of geographic variation in the structure of species interactions within local communities (for example, seed dispersal networks on insular versus mainland habitats [41] ). On shorter timescales, it is possible to show experimentally that differences in colonization rates among local habitats cause differences in community structure across a landscape [38] . For example, invertebrate predators and prey colonize experimental pond habitats at different rates. This differential colonization generates a spatial gradient in the relative abundances of species occupying different positions in a food web [38] . Variation in colonization rates across a landscape can also create spatial variation in functional structures within local food webs and the rate at which these structures develop during community assembly [39] , [43] . The results presented here suggest that effects of dispersal on community trophic structure can extend over a very large spatial scale. Our study reveals that marine predator species richness is less sensitive than prey richness to habitat isolation, and that this asymmetry causes major variation in trophic structure across Pacific coral reefs. The modelling framework developed here moves from individuals to ecosystems, illustrating how attributes of individual predator and prey larvae influence the dispersal of larval populations, and ultimately create standing variation in predator and prey species richness at an oceanic scale. These results add to a growing body of evidence suggesting that careful consideration of organismal movement may help explain the structure of the ecological communities in ecosystems across the globe. Given the suite of anthropogenic threats facing reef ecosystems [44] and top predators more generally [45] , a renewed focus on the mechanisms that govern community structure is essential. Habitat isolation and coastal length For each of the 35 focal sites, we measured the great circle distance from the centroid of the site to the nearest large potential source of larvae, defined as any landmass >10 4 km 2 (landmass size computed using a global equal area Behrmann projection) that contained coral reef habitat (alternative isolation metrics are discussed in Supplementary Methods ). We used coastal length as a measure of habitat size for each focal habitat. Coastal length was computed as the total length of the coastline of each island or set of islands at each of the 35 sites in our database. Lengths of coastlines were measured using SRTM30 PLUS bathymetry (Shuttle Radar Topography Mission) available at http://topex.ucsd.edu/WWW.html/srtm30plus.html . Species lists and assignment of trophic position Our data set included species lists from 35 islands/archipelagos with coral reef habitat and included 1,350 shallow-water reef fish species compiled in a recently published reef fish species incidence database [46] . Seventy-five percent of fish species fell into 23 families that are readily detected during surveys: Gobiidae, Labridae, Pomacentridae, Apogonidae, Serranidae, Muraenidae, Chaetodontidae, Scorpaenidae, Syngnathidae, Ophichthidae, Tripterygiidae, Callionymidae, Carangidae, Pseudochromidae, Lutjanidae, Bothidae, Pomacanthidae, Engraulidae, Soleidae, Ptereleotridae, Monacanthidae, Clupeidae and Lethrinidae. We restricted our analyses to these common families. Including species from all families did not qualitatively change our results. We defined the adult trophic position (that is, predator or prey) of each species using diet, morphology and behaviour information from fishbase ( http://www.fishbase.org ) and the primary literature, acknowledging that predation risk in coral reef fishes is high during the early life stage for nearly all species regardless of their trophic position as adults [29] . Predators were defined as species that consumed fish as ≥50% of their diets as adults. We scored each potential prey species with a palatability score. Palatability 1 is preferred prey (that is, prey that are most heavily targeted by predators); palatability 2 is occasional prey (that is, prey that are not specifically targeted by predators but are eaten occasionally); palatability 3 is rare prey that are seldom targeted by predators; and palatability 4 is non-targeted species that are avoided by predators due to anti-predator traits such as toxins, spines, morphology or behaviour. For the purposes of our analyses, prey were defined as species smaller than 20 cm in total length with palatability scores of 1 or 2. We used this designation because many marine predators are gape limited and avoid consuming heavily armed and otherwise unpalatable species [29] , [47] . We also excluded mesopredators that were categorized as both prey and predators. In Supplementary Methods , we explore the sensitivity of our results to the choice of prey designation criteria (that is, palatability and size cut-offs). Our results do not change if alternative criteria are used to define which species are considered prey. Statistical analysis As described above, we fitted functions predicted by our theoretical framework to the Pacific reef fish data. For each predicted relationship, we accounted for spatial autocorrelation by using generalized least squares to fit a set of models with different spatial autocorrelation functions. Since we had no a priori expectation about the form of the spatial autocorrelation among sites, we used AIC to compare four commonly used models of spatial autocorrelation: spherical, exponential, Gaussian and rational quadratic. For each analysis, we report statistics from the fit that included the spatial autocorrelation function yielding the lowest AIC value. The linearized model of predator–prey ratio ( R ) had the form: ln( R )= α 1 + α 2 d 2 + α 3 ln(coastal length)+Ω, where α j are regression coefficients and Ω includes spatial autocorrelation and normally distributed errors (data and model plotted in Fig. 2c ). We included coastal length (a metric of habitat size) as a predictor because habitat size is known to affect species richness, and coastal length varied among the habitats included in our analysis. The Gaussian spatial autocorrelation model had the lowest AIC (AIC=−2.5, r 2 =0.44). The analysis revealed a significant positive effect of isolation ( P =1.8 × 10 −4 ) on log (ln) predator–prey ratio and a significant negative effect of ln coastal length on ln predator–prey ratio ( P =4.2 × 10 −2 ). The linearized model of predator and prey species richness had the same form as the model of predator–prey ratio, but included interactions between predictors and trophic level to allow for the possibility that predator and prey richness were affected differently by isolation and habitat size ( Fig. 2b ). The linearized model had the form ln( S )= α 1 + α 2 d 2 + α 3 ln(coastal length)+ α 4 [ i ]+ α 5 [ i × d 2 ]+ α 6 [ i × ln(coastal length)]+Ω, where α j are regression coefficients and i is an indicator variable denoting whether each datum was a predator or prey. The statistical fit with Gaussian spatial autocorrelation had the lowest AIC (AIC=5.2, r 2 =0.78). There was a significant negative effect of isolation on ln richness ( P =1.6 × 10 −4 ) and an interaction between trophic level and isolation, such that the ln prey richness-isolation relationship declined more steeply with increasing isolation than the ln predator richness-isolation relationship ( P =9.5 × 10 −6 ; Fig. 2b ). The effect of ln coastal length on ln richness was also significant ( P =7.4 × 10 −8 ), as was the ln coastal length × trophic level interaction ( P =3.3 × 10 −2 ), which indicated that ln prey richness increased more rapidly with increasing coastal length than did ln predator richness. To display data on bivariate plots, we defined habitat size-corrected R =ln( R )−α 3 ln(coastal length), where α 3 is the fitted coastal length dependence of ln( R ). For the species richness analysis, we defined habitat size-corrected predator richness=ln( S pred )−α 3 ln(coastal length), where α 3 is the fitted coastal length dependence for predators, and we defined habitat size-corrected prey richness=ln( S prey )−( α 3 + α 6 )ln(coastal length), where ( α 3 + α 6 ) is the fitted coastal length dependence for prey. All analyses were conducted using the nlme package [48] in the R statistical programing language [49] . To determine the relationship between the number of predator and prey species at a given site, we modelled the predator richness as a function of prey richness using generalized nonlinear least squares to account for spatial autocorrelation among sites. As predicted, a power function relationship of the form, y = ax b provided a good fit to data ( Fig. 4 ). Spatial autocorrelation was best described by a spherical spatial autocorrelation model (AIC=313.3). The power function relationship between prey and predator richness accounted for most of the variation in predator richness ( r 2 =0.89, P =4.9 × 10 −16 ). How to cite this article: Stier, A. C. et al . Larval dispersal drives trophic structure across Pacific coral reefs. Nat. Commun. 5:5575 doi: 10.1038/ncomms6575 (2014).